Neural coding in a single sensory neuron controlling opposite seeking behaviours inCaenorhabditis elegans Unveiling the neural codes for intricate behaviours is a major challenge in neuroscience. The neural circuit for the temperature-seeking behaviour of Caenorhabditis elegans is an ideal system to dissect how neurons encode sensory information for the execution of behavioural output. Here we show that the temperature-sensing neuron AFD transmits both stimulatory and inhibitory neural signals to a single interneuron AIY. In this circuit, a calcium concentration threshold in AFD acts as a switch for opposing neural signals that direct the opposite behaviours. Remote control of AFD activity, using a light-driven ion pump and channel, reveals that diverse reduction levels of AFD activity can generate warm- or cold-seeking behaviour. Calcium imaging shows that AFD uses either stimulatory or inhibitory neuronal signalling onto AIY, depending on the calcium concentration threshold in AFD. Thus, dual neural regulation in opposite directions is directly coupled to behavioural inversion in the simple neural circuit. Behaviour is the ultimate consequence of orchestrated computations in neural circuits. Neuronal signalling between neurons is mainly regulated through chemical synapses and electrical gap junctions. How an individual neuron regulates complicated computation of synaptic signalling, however, remains to be fully elucidated. The thermotaxis behaviour of C. elegans is an ideal behavioural paradigm to understand the dynamics of neural circuits [1] , [2] , [3] , [4] . When wild-type C. elegans , previously cultivated at a certain temperature and with bacteria as a food source, are placed on a temperature gradient, they migrate to the previous cultivation temperature and move isothermally near that temperature [1] , [2] . The neural circuit model for thermotaxis proposed to date is one of the few circuits for the regulation of sensory behaviour [2] , [4] . After temperature is sensed by the AFD and AWC sensory neurons, the temperature information is processed in three interneurons: the AIY interneuron-mediated pathway drives warm-seeking (thermophilic) movement, the AIZ interneuron-mediated pathway drives cold-seeking (cryophilic) movement, and the counterbalancing regulation between the AIY and AIZ activities through the RIA-integrating interneuron is essential for the execution of motor output ( Fig. 1a ). 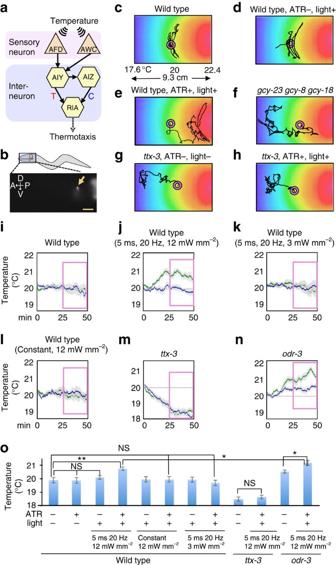Figure 1: Thermotactic phenotype of halorhodopsin-activated animals. (a) Neural circuit model for thermotaxis. Arrow indicates synaptic connection. Temperature is sensed by AFD and AWC sensory neuron. The activated AIY interneuron accelerates the movement to a temperature higher than the cultivation temperature (thermophilic drive; T), the activated AIZ accelerates the movement to a temperature lower than the cultivation temperature (cryophilic drive; C), and RIA interneuron integrates thermal signalling of 'T' and 'C'. (b) Expression of halorhodopsin fused with fluorescence protein. Arrow indicates AFD cell body. Scale bar: 25 μm. (c–h) Representative track of an animal on a temperature gradient. Adult animals, cultivated, at 20 °C were individually placed on a 9.3 cm thermal gradient between 17.6 and 22.4 °C, and were allowed to move freely for 50 min. Most wild-type animals leave striking isothermal tracks on the assay plate (c,d), whereas activation of halorhodopsin in AFD induces a thermophilic phenotype (e) that is the opposite phenotype in animals lacking guanylyl cyclases, which are essential for AFD temperature sensing (f). The temperature of the thermal gradient was measured by thermography. (i–n), Thermotaxis of 20 °C-cultivated animals. Blue indicates ATR-, light-. Green indicates ATR+, light−. Error bar indicates standard error of mean (s.e.m.). Each graph represents the average.n=15∼19 for each genotype. Halorhodopsin is expressed specifically in AFD of the animals. 25 min from 25 to 50 min (highlighted in pink) was used for comparative statistical analysis as shown ino. (o) Average temperature of animals' positions on thermal gradient during 25 min from 25 to 50 min (highlighted in pink as shown ini–n). Error bar indicates standard error of mean (s.e.m.). Single and double asterisk indicateP<0.05 and 0.01 in Dunnett test, respectively (Methods). NS, not significant (P>0.05). Figure 1: Thermotactic phenotype of halorhodopsin-activated animals. ( a ) Neural circuit model for thermotaxis. Arrow indicates synaptic connection. Temperature is sensed by AFD and AWC sensory neuron. The activated AIY interneuron accelerates the movement to a temperature higher than the cultivation temperature (thermophilic drive; T), the activated AIZ accelerates the movement to a temperature lower than the cultivation temperature (cryophilic drive; C), and RIA interneuron integrates thermal signalling of 'T' and 'C'. ( b ) Expression of halorhodopsin fused with fluorescence protein. Arrow indicates AFD cell body. Scale bar: 25 μm. ( c – h ) Representative track of an animal on a temperature gradient. Adult animals, cultivated, at 20 °C were individually placed on a 9.3 cm thermal gradient between 17.6 and 22.4 °C, and were allowed to move freely for 50 min. Most wild-type animals leave striking isothermal tracks on the assay plate ( c , d ), whereas activation of halorhodopsin in AFD induces a thermophilic phenotype ( e ) that is the opposite phenotype in animals lacking guanylyl cyclases, which are essential for AFD temperature sensing ( f ). The temperature of the thermal gradient was measured by thermography. ( i – n ), Thermotaxis of 20 °C-cultivated animals. Blue indicates ATR-, light-. Green indicates ATR+, light−. Error bar indicates standard error of mean (s.e.m.). Each graph represents the average. n =15 ∼ 19 for each genotype. Halorhodopsin is expressed specifically in AFD of the animals. 25 min from 25 to 50 min (highlighted in pink) was used for comparative statistical analysis as shown in o . ( o ) Average temperature of animals' positions on thermal gradient during 25 min from 25 to 50 min (highlighted in pink as shown in i – n ). Error bar indicates standard error of mean (s.e.m.). Single and double asterisk indicate P <0.05 and 0.01 in Dunnett test, respectively (Methods). NS, not significant ( P >0.05). Full size image The molecular mechanism of temperature sensation in C. elegans has been reported [3] . Briefly, temperature signals in the AFD and AWC neurons are transmitted through cGMP-dependent signals, such as guanylyl cyclases and a cGMP-gated channel [4] , [5] , [6] , [7] , [8] , [9] , [10] . Modulatory proteins required for temperature signalling have also been isolated. The tax-6 gene encodes the calcium-activated protein phosphatase, calcineurin [3] , [11] . The tax-6 mutant is defective in AFD and migrates towards warmer temperature than the previous cultivation temperature when placed on a temperature gradient [1] , [2] , [11] , [12] , [13] , [14] . This thermophilic abnormality of the tax-6 mutant is the opposite phenotype to the cryophilic abnormality observed in some of the AFD-ablated wild-type animals and AFD-defective mutants [2] . Previous behavioural studies therefore imply that TAX-6 acts as a negative modulator of temperature signalling and that thermophilic abnormality is caused by hyper-activation of the AFD neuron [11] , [13] . The ability to manipulate neuronal activity in a spatiotemporal manner is highly desirable to dissect the properties of neural processing. The light-driven ion pump halorhodopsin (NpHR) and the light-gated ion channel (ChR2) are suitable tools for such manipulation [15] . Halorhodopsin is a genetically encoded light-driven chloride ion pump that was originally isolated from the archaeon Natronomonas pharaonis . Excitation of halorhodopsin by yellow light rapidly activates the ion pump, allowing the influx of chloride ions in the cell, which hyperpolarizes the membrane and decreases neuronal activity [15] , [16] , [17] . Given that manipulation of neural activity using halorhodopsin has proved successful in model organisms [15] , [18] , it is likely that application of halorhodopsin to the neural circuits of C. elegans would be effective in elucidating the detailed neural code underlying neural computation and behaviour. In this study, control of neural activity using a light-driven pump and channel led us to propose that a single sensory neuron transmits both inhibitory and stimulatory neural signals to a single interneuron, and that the opposing neural signals direct opposite temperature-seeking behaviours. A combination of genetic analyses with the halorhodopsin technique demonstrated that a threshold level of intraneuronal calcium alternates the mode of neural signalling onto the downstream neuron. Our observations provide a code for the regulation of inhibitory and stimulatory neural signalling between neurons, which can generate highly variable thermotactic behaviour. Halorhodopsin activation in AFD induces thermophilic defect To elucidate the computational property of the neural circuit for thermotactic behaviour ( Fig. 1a ), we employed the light-driven chloride pump, halorhodopsin (HR). We fused the gene encoding halorhodopsin, codon-optimized for C. elegans (CeHR), with the gene encoding red fluorescent protein ( CeHR::rfp ), and constructed transgenic wild-type strains expressing CeHR::rfp specifically in the AFD thermosensory neuron ( Fig. 1b ). Using a custom-developed optical apparatus ( Supplementary Fig. S1a-d ), pulsed illumination was delivered for excitation of halorhodopsin in the AFD neurons of the transgenic animals performing thermotactic behaviour on a temperature gradient. After cultivation at 20 °C, wild-type animals expressing halorhodopsin in AFD migrated to 20 °C and moved isothermally near the previous cultivation temperature ( Fig. 1c,i blue). Similarly, the animals cultivated at 20 °C in the presence of All-Trans-Retinal (ATR), needed for activating halorhodopsin, migrated towards their cultivation temperature ( Fig. 1i green; Supplementary Fig. S2a,b ). These results indicate that ATR does not affect thermotaxis. We also verified that excitation light itself did not affect thermotaxis in animals that were cultivated without ATR ( Fig. 1d,j (ATR−, light+) and Supplementary Fig. S3 ). We found that pulsed illumination in animals cultivated with ATR induced abnormal migration towards a warmer temperature than the cultivation temperature ( Fig. 1e,j (ATR+, light+), and Supplementary Fig. S2c,d ). The thermophilic abnormalities were unexpected, because previous analysis demonstrated that cryophilic or athermotactic abnormalities were observed in animals defective in AFD function, such as AFD-ablated wild-type animals [2] and the mutant animals lacking the three guanylyl cyclases GCY-23, GCY-8 and GCY-18 that are essential for temperature sensing in AFD ( Fig. 1f ) [6] . Low-power pulsed light did not affect thermotaxis ( Fig. 1k ). Likewise, constant light did not affect thermotaxis ( Fig. 1l and Supplementary Fig. S2d ), implying that the continuous illumination desensitized halorhodopsin, as previously reported [15] . These results indicate that abnormal migration to a warmer temperature than the cultivation temperature is caused by pulsed excitation of halorhodopsin in AFD. Halorhodopsin activation in AFD affects AIY neural pathway The temperature-sensing neuron AFD connects to its downstream interneuron AIY with chemical synapses, and the AFD–AIY neural pathway is important for thermophilic movement ( Fig. 1a ) [2] . To investigate whether the thermophilic abnormality observed upon activation of halorhodopsin in AFD is ascribed to abnormal temperature signalling through the AFD–AIY neural pathway, we analysed mutant animals defective in the component neurons of the thermotaxis neural circuit ( Fig. 1g,h,m–o ). Activation of halorhodopsin in AFD of ttx-3 mutants exhibiting aberrant AIY development caused cryophilic abnormalities ( Fig. 1h,m (ATR+, light+)), similar to that of ttx-3 mutants without halorhodopsin activation ( Fig. 1g,m (ATR−, light−)) [19] . These results suggest that activation of halorhodopsin in AFD directly or indirectly affects the AIY-mediated neural pathway. AIY is a postsynaptic interneuron for two temperature-sensing neurons, AFD and AWC ( Fig. 1a ) [2] , [4] . The odr-3 gene encodes the trimetric guanine nucleotide-binding protein (G protein) alpha subunit ODR-3 that is a key molecule for temperature sensing in AWC, and the odr-3 mutant shows a weak thermophilic abnormality ( Fig. 1n (ATR−, light−)) [4] , [20] . It is possible that the thermophilic abnormality observed by the activation of halorhodopsin in AFD of wild-type animals is caused by indirect disruption of AWC through an unidentified neural pathway, such as the gap junction network [21] . To eliminate this possibility, we activated halorhodopsin in AFD of the odr-3 mutant animals. Activation of halorhodopsin in AFD of the odr-3 mutant caused a stronger thermophilic abnormality than that of the naive odr-3 mutant ( Fig. 1n green), implying that the halorhodopsin-induced thermophilic abnormality is independent of the AWC-dependent pathway. We next directly monitored AWC activity as a temperature-evoked calcium concentration change, using the genetically encoded calcium indicator cameleon [22] . We found that activation of halorhodopsin in AFD of wild-type animals did not affect the calcium concentration change in AWC upon temperature change ( Fig. 2g ). Taken together, these results suggest that activation of halorhodopsin in AFD affects the AFD–AIY neural pathway essential for thermophilic movement ( Fig. 1a ). 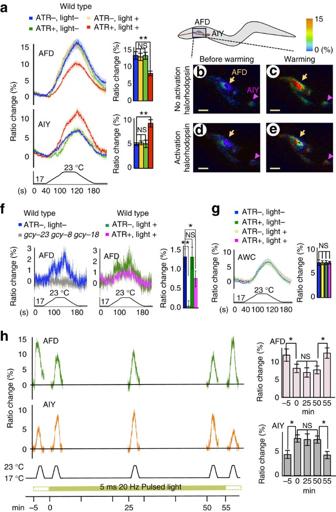Figure 2: Optical recording of neural activity in the thermotaxis neural circuit in halorhodopsin-activated wild-type animal. (a)In vivocalcium imaging. Relative changes in the intracellular calcium concentration were measured as changes in the YFP/CFP fluorescence of the cameleon protein ratio22(Ratio change). Temperature change along time is shown at the bottom of the graph. 'Light +' indicates 5 ms 20 Hz pulsed-light for activating halorhodopsin. Bar graph, average ratio change during 20 s from 100 to 120 s. The colour key for bar graph is the same as that for the corresponding response curve. Each graph represents the average response to temperature stimuli. Error bar indicates s.e.m. Double asterisk indicatesP<0.01 in Dunnett test. NS, not significant.n=17–22. (b–e), A schematic diagram of an AFD and AIY in the head, and corresponding pseudocolour images depicting the fluorescence ratio of cameleon before (b,d) and during temperature changes (c,e). Arrow and arrowhead indicate AFD cell body and AIY neurite, respectively. Scale bar: 10 μm. (f)In vivomembrane voltage imaging of AFD. Relative changes in the intracellular membrane voltage were measured as changes in the mKOk/mUKG fluorescence of the mermaid protein ratio29. Bar graph, average ratio change during 90 s from 60 to 150 s. Error bar indicates s.e.m. Single asterisk indicatesP<0.05 in Dunnett test. NS, not significant.n=27–38. (g) Calcium imaging of AWC in wild-type animals expressing halorhodopsin in AFD. Activation of halorhodopsin in AFD did not affect temperature-evoked calcium concentration changes in AWC. Bar graph, average ratio change during 20 second from 100 to 120 s. Error bar indicates s.e.m. NS, not significant in Dunnett test.n=11∼14. (h) Time course calcium imaging of AFD and AIY. Pulsed-light (5 ms, 20 Hz, 12 mW mm−2) was illuminated for 50 min. Each graph represents the average. Error bar indicates s.e.m. Single asterisk indicatesP<0.05 in Dunnett test. NS, not significant.n=10. Figure 2: Optical recording of neural activity in the thermotaxis neural circuit in halorhodopsin-activated wild-type animal. ( a ) In vivo calcium imaging. Relative changes in the intracellular calcium concentration were measured as changes in the YFP/CFP fluorescence of the cameleon protein ratio [22] (Ratio change). Temperature change along time is shown at the bottom of the graph. 'Light +' indicates 5 ms 20 Hz pulsed-light for activating halorhodopsin. Bar graph, average ratio change during 20 s from 100 to 120 s. The colour key for bar graph is the same as that for the corresponding response curve. Each graph represents the average response to temperature stimuli. Error bar indicates s.e.m. Double asterisk indicates P <0.01 in Dunnett test. NS, not significant. n =17–22. ( b – e ), A schematic diagram of an AFD and AIY in the head, and corresponding pseudocolour images depicting the fluorescence ratio of cameleon before ( b , d ) and during temperature changes ( c , e ). Arrow and arrowhead indicate AFD cell body and AIY neurite, respectively. Scale bar: 10 μm. ( f ) In vivo membrane voltage imaging of AFD. Relative changes in the intracellular membrane voltage were measured as changes in the mKO k /mUKG fluorescence of the mermaid protein ratio [29] . Bar graph, average ratio change during 90 s from 60 to 150 s. Error bar indicates s.e.m. Single asterisk indicates P <0.05 in Dunnett test. NS, not significant. n =27–38. ( g ) Calcium imaging of AWC in wild-type animals expressing halorhodopsin in AFD. Activation of halorhodopsin in AFD did not affect temperature-evoked calcium concentration changes in AWC. Bar graph, average ratio change during 20 second from 100 to 120 s. Error bar indicates s.e.m. NS, not significant in Dunnett test. n =11 ∼ 14. ( h ) Time course calcium imaging of AFD and AIY. Pulsed-light (5 ms, 20 Hz, 12 mW mm −2 ) was illuminated for 50 min. Each graph represents the average. Error bar indicates s.e.m. Single asterisk indicates P <0.05 in Dunnett test. NS, not significant. n =10. Full size image AFD transmits diverse neural signals onto AIY The thermophilic abnormality induced by activating halorhodopsin in AFD of wild-type animals is opposite to the cryophilic abnormality observed in animals lacking AFD or AIY ( Fig. 1e,f ). To quantify this neural activity, we monitored temperature-evoked changes in the intracellular calcium concentration in intact AFD and AIY neurons, using the calcium indicator cameleon [22] . Sodium-dependent action potentials are thought to be lacking in C. elegans neurons, and, instead, voltage-gated calcium channels are rapidly activated in the neurons [8] , [10] , [23] , [24] , [25] , [26] , [27] , [28] . Optical recording of calcium concentration in previous studies and the current study revealed that the calcium concentration in AFD of wild-type animals increased upon temperature change ( Fig. 2a–c ) [9] , [10] . Pulsed excitation of halorhodopsin in AFD partially reduced the temperature-evoked calcium concentration changes in AFD ( Fig. 2a,d,e ). Using another fluorescent protein, mermaid, which acts as a membrane voltage indicator [29] , we confirmed that activation of halorhodopsin in AFD induced hyperpolarization of AFD ( Fig. 2f ). These optical analyses suggest that halorhodopsin can reduce the neuronal activity of AFD. The calcium concentration change in AFD was followed by an increase in the calcium concentration in AIY ( Fig. 2a–c ) [10] , [30] . Temperature information from AFD is thus conveyed to AIY through a stimulatory neural signal [10] , [30] . However, pulsed excitation of halorhodopsin in AFD significantly enhanced the calcium concentration change in AIY upon temperature change, even though AFD activity itself was partially reduced ( Fig. 2a,d–f ; Supplementary Movies 1 , 2 ). This phenomenon was observed for at least 50 min, namely throughout the pulsed illumination for the excitation of halorhodopsin ( Fig. 2h ). These results are consistent with the model in which AFD transmits diverse neural signals onto the single interneuron AIY. Calcium concentration changes in AFD diversely regulate AIY To investigate the relationship between AFD activity and AIY activity, we simultaneously measured calcium concentration changes in AFD and AIY in various mutants defective in AFD temperature signalling. We first analysed mutant animals showing thermophilic abnormalities that were similar to the halorhodopsin-induced behavioural phenotype in wild-type animals. The mutants with a partially impaired microvillus structure of the AFD sensory endings due to the defect in the glial sheath cell surrounding the AFD dendrite, exhibited thermophilic abnormalities ( Fig. 3d ) [31] . We demonstrated that the calcium concentration in AIY of such glial cell mutants notably increased in response to thermal stimuli ( Fig. 4a,b,g AIY), whereas the thermal response of AFD itself was partially reduced ( Fig. 4a,b,g AFD). Similar abnormal calcium concentration changes in both AFD and AIY were observed in another thermophilic mutant, tax-6 calcineurin ( Figs 3b,e and 4c ), which has impaired modulation of AFD temperature sensation [11] . Thermophilic abnormalities and hyper-activation of AIY in tax-6 mutants were both slightly enhanced by the activation of halorhodopsin in AFD ( Figs 3f and 4c ). Baseline levels of the ratio before warming were similar between the wild-type animals and the mutants, suggesting that the resting calcium levels are normal in the mutants ( Fig. 4h ). These results are consistent with a hypothesis that the partially defective responsiveness of AFD to thermal stimuli causes hyper activation of AIY, thereby generating the thermophilic abnormality. 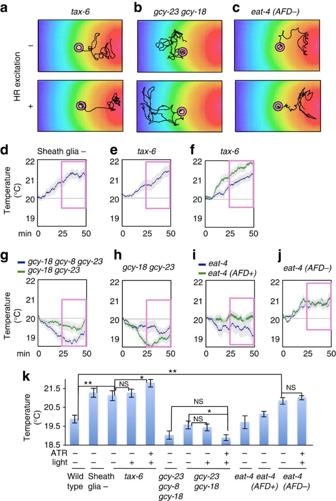Figure 3: Thermotaxis of halorhodopsin-activated mutant animals. (a–c) Representative tracks of 20 °C-cultivated animals expressing halorhodopsin in AFD. Adult animals were individually placed on a 9.3 cm thermal gradient between 17.6 and 22.4 °C, and were allowed to move freely for 50 min. (d,e) Thermotaxis of 20 °C-cultivated thermophilic mutant animals. 25 min from 25 to 50 min (highlighted in pink) was used for comparative statistical analysis as shown in k. Each graph represents the average. Error bar indicates s.e.m.n=12 (d) and 19 (e). (f) Thermotaxis of 20 °C-cultivatedtax-6mutant animals. Blue indicates ATR−, light+. Green indicates ATR+, light+. 5 ms 20 Hz pulsed-light (12 mW mm−2) was illuminated for activating halorhodopsin. Error bar indicates s.e.m.n=14 for each graph. (g) Thermotaxis of 20 °C-cultivatedgcy-18 gcy-8 gcy-23andgcy-18 gcy-23animals. Blue indicates ATR-, light+. Green indicates ATR+, light+. n=15 for blue and 19 for green. (h) Thermotaxis of 20 °C-cultivatedgcy-18 gcy-23mutant animals. Blue indicates ATR-, light-. Green indicates ATR+, light+. 5 ms 20 Hz pulsed-light (12 mW mm−2) was illuminated for activating halorhodopsin. Error bar indicates s.e.m.n=16 for blue and 14 for green. (i) Summary for thermotaxis of 20 °C-cultivatedeat-4mutant animals. Each graph represents the average. Theeat-4mutant shows athermotactic abnormality (blue), which was restored by expressing EAT-4 in AFD, AWC and RIA in the thermotaxis neural circuit (green), as reported recently34. Error bar indicates s.e.m.n=14 for each genotype. (j) Thermotaxis of 20 °C-cultivated animals. Blue indicates ATR−, light−. Green indicates ATR+, light+. Expression of EAT-4 in AWC and RIA ofeat-4mutant induced thermophilic abnormality (blue), where malfunctions of EAT-4 in AWC and RIA are restored but EAT-4 in AFD remains to be impaired. 5 ms 20 Hz pulsed-light (12 mW mm−2) was illuminated for activating halorhodopsin. Error bar indicates s.e.m.n=14 for blue and 13 for green. (k) Average temperature in each time point of moving animals on thermal gradient during 25 min from 25 to 50 min (highlighted in pink as shown ind–j). Error bar indicates s.e.m. Single and double asterisk indicateP<0.05 and 0.01 in Dunnett test, respectively. NS, not significant. Figure 3: Thermotaxis of halorhodopsin-activated mutant animals. ( a – c ) Representative tracks of 20 °C-cultivated animals expressing halorhodopsin in AFD. Adult animals were individually placed on a 9.3 cm thermal gradient between 17.6 and 22.4 °C, and were allowed to move freely for 50 min. ( d , e ) Thermotaxis of 20 °C-cultivated thermophilic mutant animals. 25 min from 25 to 50 min (highlighted in pink) was used for comparative statistical analysis as shown in k. Each graph represents the average. Error bar indicates s.e.m. n =12 ( d ) and 19 ( e ). ( f ) Thermotaxis of 20 °C-cultivated tax-6 mutant animals. Blue indicates ATR−, light+. Green indicates ATR+, light+. 5 ms 20 Hz pulsed-light (12 mW mm −2 ) was illuminated for activating halorhodopsin. Error bar indicates s.e.m. n =14 for each graph. ( g ) Thermotaxis of 20 °C-cultivated gcy-18 gcy-8 gcy-23 and gcy-18 gcy-23 animals. Blue indicates ATR-, light+. Green indicates ATR+, light+. n=15 for blue and 19 for green. ( h ) Thermotaxis of 20 °C-cultivated gcy-18 gcy-23 mutant animals. Blue indicates ATR-, light-. Green indicates ATR+, light+. 5 ms 20 Hz pulsed-light (12 mW mm −2 ) was illuminated for activating halorhodopsin. Error bar indicates s.e.m. n =16 for blue and 14 for green. ( i ) Summary for thermotaxis of 20 °C-cultivated eat-4 mutant animals. Each graph represents the average. The eat-4 mutant shows athermotactic abnormality (blue), which was restored by expressing EAT-4 in AFD, AWC and RIA in the thermotaxis neural circuit (green), as reported recently [34] . Error bar indicates s.e.m. n =14 for each genotype. ( j ) Thermotaxis of 20 °C-cultivated animals. Blue indicates ATR−, light−. Green indicates ATR+, light+. Expression of EAT-4 in AWC and RIA of eat-4 mutant induced thermophilic abnormality (blue), where malfunctions of EAT-4 in AWC and RIA are restored but EAT-4 in AFD remains to be impaired. 5 ms 20 Hz pulsed-light (12 mW mm −2 ) was illuminated for activating halorhodopsin. Error bar indicates s.e.m. n =14 for blue and 13 for green. ( k ) Average temperature in each time point of moving animals on thermal gradient during 25 min from 25 to 50 min (highlighted in pink as shown in d – j ). Error bar indicates s.e.m. Single and double asterisk indicate P <0.05 and 0.01 in Dunnett test, respectively. NS, not significant. 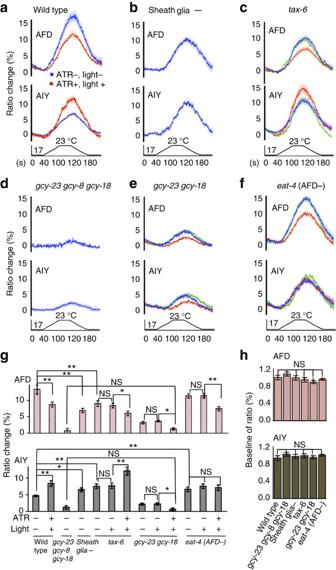Figure 4: Calcium imaging in halorhodopsin-activated mutant animals with impairment in AFD temperature signalling. (a–f) Calcium imaging of AFD and AIY neurons in animals subjected to warming and cooling. Blue, green and red indicate [ATR−, light−], [ATR−, light+] and [ATR+, light+], respectively (c,e,f). A partial decrease in AFD activity increased AIY activity in thermophilic mutant animals (b,cblue). Activation of halorhodopsin in AFD reduced AFD activity, but did not affect AIY activity in theeat-4(AFD-) mutants (f red). Error bar indicates s.e.m. Each graph represents the average.n=17∼20. 'Light +' indicates 5 ms 20 Hz pulsed-light (12 mW mm−2) for activation of halorhodopsin. (g) Average ratio change during 20 s between 100 and 120 s after delivering temperature change. Error bar indicates s.e.m. Single and double asterisk indicateP< 0.05 and 0.01 in Dunnett test, respectively. NS, not significant (P>0.05). (h) Baseline levels of the ratio between YFP and CFP of cameleon protein in AFD and AIY before warming. Error bar indicates s.e.m. Each graph represents the average.n=18∼22. Full size image Figure 4: Calcium imaging in halorhodopsin-activated mutant animals with impairment in AFD temperature signalling. ( a – f ) Calcium imaging of AFD and AIY neurons in animals subjected to warming and cooling. Blue, green and red indicate [ATR−, light−], [ATR−, light+] and [ATR+, light+], respectively ( c , e , f ). A partial decrease in AFD activity increased AIY activity in thermophilic mutant animals ( b , c blue). Activation of halorhodopsin in AFD reduced AFD activity, but did not affect AIY activity in the eat-4 (AFD-) mutants (f red). Error bar indicates s.e.m. Each graph represents the average. n =17 ∼ 20. 'Light +' indicates 5 ms 20 Hz pulsed-light (12 mW mm −2 ) for activation of halorhodopsin. ( g ) Average ratio change during 20 s between 100 and 120 s after delivering temperature change. Error bar indicates s.e.m. Single and double asterisk indicate P < 0.05 and 0.01 in Dunnett test, respectively. NS, not significant ( P >0.05). ( h ) Baseline levels of the ratio between YFP and CFP of cameleon protein in AFD and AIY before warming. Error bar indicates s.e.m. Each graph represents the average. n =18 ∼ 22. Full size image We next analysed cryophilic mutants that are impaired in AFD temperature signalling. Three guanylyl cyclases, GCY-23, GCY-8 and GCY-18, are essential for temperature input at the sensory endings of AFD [6] , [8] , [32] . The gcy-23 gcy-8 gcy-18 triple mutant, which showed a severe cryophilic abnormality in this study ( Figs 1f and 3g,k ) failed to show calcium concentration changes in both AFD and AIY in response to thermal stimuli ( Fig. 4d ). gcy-23 gcy-18 double mutant animals showed a weaker cryophilic abnormality ( Fig. 3b,h blue), as previously reported [6] . Calcium imaging revealed that activation of halorhodopsin in AFD of the gcy-23 gcy-18 mutant reduced the calcium concentrations in both AFD and AIY ( Fig. 4e,g ), and enhanced the severity of the cryophilic abnormality ( Fig. 3b,h ). These phenotypes are similar to the phenotypes of the gcy-23 gcy-8 gcy-18 triple mutants ( Figs 1f , 3g and 4d ). Thus, a strong decrease in the calcium concentration in AFD in response to thermal stimuli impairs neuronal activation of AIY. To investigate how the AIY responses are dependent on the AFD responses, we conducted a systematic dose-response experiment using different degrees of temperature increment and decrement ( Fig. 5 ). Weak increments in calcium concentration in AFD ( Fig. 5b blue, c blue, f blue, g and h) increased the calcium concentrations in AIY. A small reduction in the AFD response from its maximum response achieved by temperature increment from 17 to 24.5 °C ( Fig. 5e blue) induced the strongest response in AIY, which is reminiscent of the calcium concentration changes in the thermophilic mutants ( Fig. 4b,c ). By contrast, the strongest increment in calcium concentration in AFD, achieved by temperature increment from 17 to 23 °C ( Fig. 5d (blue)), suppressed the AIY responses. The small AFD response achieved by temperature increment from 17 to 18.5 °C ( Fig. 5a blue), 17–20 °C ( Fig. 5b blue), 17–21.5 °C ( Fig. 5c blue), or 17–26 °C ( Fig. 5f blue) was sufficiently suppressed by activation of halorhodopsin in AFD ( Fig. 5a–c,f magenta), which in turn reduced AIY responses rather than enhanced them ( Fig. 5d,e magenta). 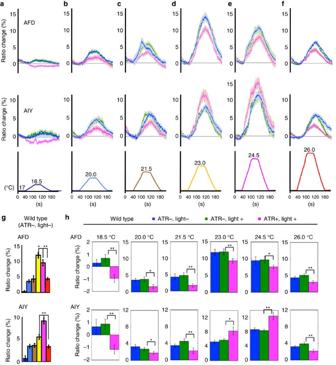Figure 5: Relationship between increasing AFD responses and AIY responses. (a–f) Calcium imaging of AFD and AIY neurons of wild-type animals in a systematic dose-response experiment using different degrees of temperature increment and decrement. Blue, green and magenta indicate [ATR−, light−], [ATR−, light+] and [ATR+, light+], respectively. Temperature change along time is shown at the bottom of the graph. halorhodopsin was expressed in AFD specifically. 'Light +' indicates 5 ms 20 Hz pulsed-light (12 mW mm−2) for activation of halorhodopsin. Error bar indicates s.e.m. Each graph represents the average.n=13∼22. (g) Average ratio change of wild-type animals (ATR−, light−) (a–f) during 20 s from 100 to 120 s after starting temperature change. The colour key for bar graph is the same as that for the corresponding temperature curve shown at the bottom of the grapha–f. (h) The average ratio change of the respective animals (a–f) is shown during the 20-s period from 100 to 120 s after starting the temperature change. The colour key for the bar graph is the same as that for the corresponding response curve shown ina–f. The error bars indicate s.e.m.n=13–22. Single and double asterisks indicateP<0.05 andP<0.01, respectively, by the Dunnett test. 'Light +' indicates 5 ms 20 Hz pulsed-light (12 mW mm−2) for activation of halorhodopsin. Figure 5: Relationship between increasing AFD responses and AIY responses. ( a – f ) Calcium imaging of AFD and AIY neurons of wild-type animals in a systematic dose-response experiment using different degrees of temperature increment and decrement. Blue, green and magenta indicate [ATR−, light−], [ATR−, light+] and [ATR+, light+], respectively. Temperature change along time is shown at the bottom of the graph. halorhodopsin was expressed in AFD specifically. 'Light +' indicates 5 ms 20 Hz pulsed-light (12 mW mm −2 ) for activation of halorhodopsin. Error bar indicates s.e.m. Each graph represents the average. n =13 ∼ 22. ( g ) Average ratio change of wild-type animals (ATR−, light−) ( a – f ) during 20 s from 100 to 120 s after starting temperature change. The colour key for bar graph is the same as that for the corresponding temperature curve shown at the bottom of the graph a – f . ( h ) The average ratio change of the respective animals ( a – f ) is shown during the 20-s period from 100 to 120 s after starting the temperature change. The colour key for the bar graph is the same as that for the corresponding response curve shown in a – f . The error bars indicate s.e.m. n =13–22. Single and double asterisks indicate P <0.05 and P <0.01, respectively, by the Dunnett test. 'Light +' indicates 5 ms 20 Hz pulsed-light (12 mW mm −2 ) for activation of halorhodopsin. Full size image Altogether, these data suggest that the calcium concentration changes in AFD in response to thermal stimuli diversely regulate neural signalling from AFD to AIY. Halorhodopsin effect interrupts inhibitory signalling on AIY Our behavioural and calcium imaging analyses enabled us to hypothesize that the thermophilic abnormality induced by pulsed excitation of halorhodopsin in AFD of wild-type animals is caused by a reduction in the neural signalling to AIY. To investigate this further, we activated halorhodopsin in AFD of mutant animals that are specifically defective in inhibitory synaptic signalling in AFD. EAT-4, a vesicular glutamate transporter, is a key molecule for the uptake of glutamate into synaptic vesicles ( Fig. 3i ) [33] . A recent analysis showed that EAT-4 is required for inhibitory synaptic transmission in the AFD–AIY circuit, and a lack of EAT-4 function in AFD synapses increased the calcium concentration change in AIY in response to thermal stimuli ( Fig. 4f blue,g ), thereby inducing a thermophilic abnormality ( Fig. 3j blue, k) [34] . These abnormalities are similar to the phenotype of wild-type animals with activated halorhodopsin in AFD ( Figs 1e,j green and 2a red). To analyse whether pulsed excitation of halorhodopsin in AFD affects EAT-4-mediated inhibitory synaptic transmission, we activated halorhodopsin in AFD of mutant animals lacking EAT-4 in AFD ( eat-4 (AFD −) mutant) ( Figs 3c,j and 4f ). The thermophilic abnormality of the eat-4 (AFD −) mutant was not affected by activation of halorhodopsin in AFD ( Fig. 3j green). Moreover, the calcium concentration in AIY of eat-4 (AFD −) mutants in response to temperature changes was not enhanced by activation of halorhodopsin in AFD, although the calcium concentration change in AFD itself was reduced ( Fig. 4f red). These results are consistent with a model that pulsed excitation of halorhodopsin in AFD of wild-type animals interrupts EAT-4-dependent inhibitory neural signalling on AIY. Exploration of the neural code for neural processing is an important challenge in neuroscience. In this study, combined analysis using optical control of neuronal activity and genetic approaches suggested that calcium concentration changes in a single sensory neuron in response to temperature stimuli may act as a switch between inhibitory and stimulatory neural signals to a single interneuron, thus controlling opposing temperature preferences. Previous reports have described that mutant animals defective in the temperature-sensing neuron AFD show various thermotactic abnormalities, such as cryophilic, thermophilic and athermotactic phenotypes [3] , [6] , [7] , [11] , [13] , [35] . Cryophilic abnormalities are observed in wild-type animals lacking the AFD or AIY neurons and in mutant animals lacking guanylyl cyclases (GCY-23, GCY-8 and GCY-18) essential for temperature sensory input ( Figs 1f and 3b,g ) [2] , [6] . Thermophilic abnormality is observed in mutant animals lacking TAX-6 calcineurin function in AFD ( Fig. 3a,e ) [11] . Because the thermophilic phenotype is opposite to the cryophilic phenotype often observed in AFD-ablated animals, we previously hypothesized that the thermophilic abnormality of tax-6 mutants is caused by hyper-activation of AFD [11] , [13] . Nevertheless, the control of neural activity with halorhodopsin in combination with the use of calcium imaging and membrane voltage imaging techniques revealed that the thermophilic abnormality is caused by a partial reduction of AFD activity in response to thermal stimuli ( Figs 1e,j and 2a,f ). Although AFD activity is reduced in these animals, the AIY calcium concentration is increased ( Fig. 2a ). Thus, the weak reduction in AFD calcium concentration in response to temperature stimuli may cause hyper activation of the AIY interneuron, which is important for thermophilic movement ( Fig. 1a ). As recently revealed, EAT-4 (VGLUT) is required for inhibitory glutamate synaptic signalling in the AFD–AIY circuit, in which glutamate opens the chloride channel GLC-3 in AIY [34] . Mutant animals lacking EAT-4 in AFD or GLC-3 in AIY exhibited thermophilic abnormalities that are caused by an aberrant hyper-temperature responsiveness of AIY [34] . Activation of halorhodopsin in AFD did not influence the thermophilic abnormality or the hyper-temperature response of AIY in the eat-4 (VGLUT) mutant ( Figs 3j green 4f red). Namely, partial reduction of AFD activity due to pulsed excitation of halorhodopsin may reduce at least EAT-4-dependent inhibitory neural signalling ( Fig. 6a,c ), whereby leading to a relatively more active state of stimulatory signalling onto AIY, which is essential for the thermophilic phenotype. 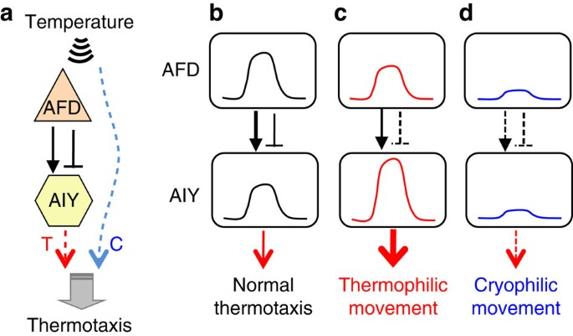Figure 6: A model for neural regulation in AFD–AIY circuit. (a) A model for neural computation of stimulatory and inhibitory neural signal controlling opposite thermotactic behaviour. Although it is likely that more complicated systems control diverse neural signalling, we describe here a plausible simple neural model. (b) Wiring diagram of stimulatory and inhibitory neural signalling in AFD–AIY circuit. Black arrow or inverted-'T' between AFD and AIY indicate stimulatory or inhibitory neural signalling, respectively. 'T' and 'C' indicate thermophilic and cryophilic driving signal, respectively. Dotted-blue line indicates AIZ-mediated cryophilic driving pathway as described inFigure 1a. Neural calculation in AFD and AIY is essential for thermophilic movement. A strong thermosensory signal activates both stimulatory and inhibitory neural signalling to AIY, inducing a weak activation of AIY. (c) A weak sensory signal induces relatively more active state of stimulatory signalling, leading to a strong activation of AIY important for thermophilic drive. (d) A lack of sensory signal eliminates AIY activity, then AIY-independent cryophilic driving signal generates cryophilic movement. The width of arrow indicates the strength of signal, and dotted arrows indicate weakness of signal. Figure 6: A model for neural regulation in AFD–AIY circuit. ( a ) A model for neural computation of stimulatory and inhibitory neural signal controlling opposite thermotactic behaviour. Although it is likely that more complicated systems control diverse neural signalling, we describe here a plausible simple neural model. ( b ) Wiring diagram of stimulatory and inhibitory neural signalling in AFD–AIY circuit. Black arrow or inverted-'T' between AFD and AIY indicate stimulatory or inhibitory neural signalling, respectively. 'T' and 'C' indicate thermophilic and cryophilic driving signal, respectively. Dotted-blue line indicates AIZ-mediated cryophilic driving pathway as described in Figure 1a . Neural calculation in AFD and AIY is essential for thermophilic movement. A strong thermosensory signal activates both stimulatory and inhibitory neural signalling to AIY, inducing a weak activation of AIY. ( c ) A weak sensory signal induces relatively more active state of stimulatory signalling, leading to a strong activation of AIY important for thermophilic drive. ( d ) A lack of sensory signal eliminates AIY activity, then AIY-independent cryophilic driving signal generates cryophilic movement. The width of arrow indicates the strength of signal, and dotted arrows indicate weakness of signal. Full size image To investigate the molecular mechanisms of the stimulatory signalling in the AFD–AIY circuit, we used mutant animals defective in stimulatory neural signalling such as acetylcholine, monoamine and neuropeptide ( Supplementary Fig. S4 ). The calcium concentration changes in AFD and AIY in such mutants were apparently normal in response to thermal stimuli from 17 to 23 °C ( Supplementary Fig. S4 ), implying that another neurotransmitter, multiple neurotransmitters or unidentified electrical gap junction are involved in the stimulatory signalling. Based on our results in this study, we provide a model for regulation of neural signalling in the AFD-AIY circuit and behavioural conversion ( Fig. 6a,b ). Large calcium concentration changes in AFD in response to thermal stimuli activate both stimulatory and inhibitory neural signalling to AIY, then inducing a relatively weak increment in the calcium concentration in AIY ( Fig. 6b ). Small calcium concentration changes in AFD induces a more active state of stimulatory neural signalling to AIY, leading to a relatively large increment in calcium concentration in AIY, important for thermophilic movement ( Fig. 6c ). A complete or virtually complete loss of sensory signal eliminates both stimulatory and inhibitory neural signalling, in which an AIY-independent cryophilic driving signal generates cryophilic movement ( Fig. 6d ). It is also likely that more complicated neural systems control diverse neural signalling in the AFD–AIY circuit, although we describe here a plausible simple neural model. It is possible that the pulsed excitation of halorhodopsin in AFD induced an unexpected-event in AIY, such as pulsed rebound excitation. We, however, showed that a small decrement in AFD activity induced an increment in AIY activity in intact wild-type animals not expressing halorhodopsin ( Fig. 5d,e,g ), and that a small decrement in AFD activity induced an increment in AIY activity in thermophilic mutant animals not expressing halorhodopsin ( Fig. 4b,c ). These results are consistent with a model that a threshold of AFD activity diversely regulates AIY activity ( Fig. 6 ). A recent report described that the odorant-sensing neuron AWC transmits inhibitory and stimulatory signals to the AIA interneuron [21] . Analysis of the mutant animals containing a mutation in guanylyl cyclase GCY-28, which is localized to the AWC axon, demonstrated that the AWC neuron can switch modes of neurotransmission for attractive and repulsive behaviour to an odorant [36] . Although this neural regulation system is similar to the system found in the present study, our findings provide a novel conceptual model of intraneuronal computation in a single sensory neuron for controlling opposing stimulatory and inhibitory neural signalling onto a single interneuron ( Fig. 6b–d ). This neural coding should offer an efficient regulatory mechanism to control the sensitivity of local sensory neural circuits. Further studies on this circuit should shed light on other characteristics of neural coding and neural processing that regulate behavioural outputs. Strains We used the following C. elegans strains: wild-type N2 Bristol, MT3644 odr-3(n1605) V, IK598 gcy-23(nj37) gcy-8(oy44) gcy-18(nj38) IV, gcy-23(nj37) gcy-18(nj38) IV, ttx-3(ks5) X, tax-6(db60) IV, eat-4(ky5) III, nsIs113[F16F9.3p::DT-A(G53E)] as a glial sheath cell defective animal, lite-1(xu7) X, unc-17(e245) IV, egl-3(n729) V, cat-1(e1111) X. Behavioural assays Single animal thermotaxis assay was performed with a thermal gradient on a microscope stage. A stable thermal gradient (0.54 °C cm −1 ) was established on a 14-cm-long glass plate containing indium tin oxide (ITO) in a custom-made temperature-gradient control system, MATS-OTORG-CU (TOKAI HIT). To establish the temperature gradient, a constant electrical current (183–206 mA) was passed and a voltage (21–23.8 V) maintained through the ITO using a current-voltage controller PMC35-0.5A (KIKUSUI). To make a thermal gradient ranging from 17.6 to 22.4 °C, cooling water (10–10.8 °C) was circulated under the ITO glass using an RTE-10 pumped water bath (NESLAB), in which the temperature of the water bath was 7.2–8 °C. Water inflow and outflow were constantly maintained at 200 ml min −1 using a Flowmeter 400CCM (KOFLOC). A thermotaxis assay (TTX) plate was prepared, consisting of a 14 cm (in length)×10 cm (in width)×1.45 cm (in height) plastic dish containing 18 ml of TTX medium with 2% agar, and was placed on the ITO glass plate on the stage of MVX-10 microscope (Olympus, Japan). The agar medium on the plastic dish was cut into 9.3 cm (in length)×6 cm (in width) rectangle, such that a temperature gradient could be established along the 9.3 cm agar surface. The top-left corner of the agar rectangle was positioned 2.1 and 0.4 cm from the top edge and the left edge of the plastic dish, respectively. A thin glass plate (13.5 cm×9.5 cm, 0.1 cm thick) was placed between the bottom of the agar rectangle and the ITO glass. The centre of the 9.3 cm-long agar surface was adjusted to 20 °C and was maintained for 30 min before a linear thermal gradient ranging from approximately 17.6 to 22.4 °C was established on the agar surface. The microscope combined with the apparatus creating thermal gradients was covered with a plastic chamber in order to maintain the temperature surrounding the thermal gradient. The temperature in the chamber was set to 21–22 °C. The temperature of the thermal gradient was measured by thermography using a TS9230 thermo tracer (NEC AVIO). To calibrate the thermal gradient, the temperature of left-right ends of the agar plate and the temperature of the water flowing under the ITO were constantly monitored using a thermistor thermometer SG4115 (ANRITSU). The TTX plate was covered with polyethylene cling-film to prevent the agar plate from drying, and to transmit infrared light for the thermography. Uncrowded and well-fed animals were used for the TTX assay. A single adult animal was placed on a 6-cm plate containing 14 ml of nematode growth medium with 2% agar, on which Escherichia coli OP50 was seeded; the animal and its progeny were cultured for about 85–90 h at 20 °C. The L4 larvae (12–24 animals per 6-cm plate) were cultured with food ( E. coli strain OP50) at the designated temperature for 8–12 h under uncrowded conditions. Fully matured, actively egg-laying adult animals were allowed to move freely for 50 min on the assay plate. Population thermotaxis assay was performed as follows. A stable, linear thermal gradient was established on a 60-cm long aluminum platform, one end of which was placed in a water bath at 5 °C and the opposite end in a water bath at 35 °C. TTX plate (14 cm×10 cm, 1.45 cm in height) containing 18 ml of TTX medium with 2% agar was placed on the aluminum plate such that temperature gradient could be established along the agar surface of 14 cm long. A thin aluminum plate (13.5 cm×9.5 cm, 0.1 cm thick) was placed in the space between the bottom of the TTX plate and the aluminum platform, and the extra space was filled with water to increase thermal conductivity as much as possible. The centre of the 14 cm long-agar surface in TTX plate was adjusted at 20 degree and the TTX plate was maintained for 20 min before a linear thermal gradient ranging from approximately 17–23 °C was established on the agar surface. Uncrowded and well-fed animals were used for the TTX assay. A single adult animal was placed on a 6-cm plate containing 14 ml of nematode growth medium with 2% agar, on which E. coli OP50 was seeded; the animal and its progeny were cultured for about 85–90 h at 20 °C. The animals were collected with 1 ml of NG buffer (0.3% NaCl, 1 mM CaCl 2 , 1 mM MgSO 4 , 25 mM potassium phosphate, pH 6.0) kept at 20 °C and were washed once with NG buffer at 20 °C. These steps were carried out within 4 min in a water bath maintained at 20 °C. Approximately 80–200 animals were placed at the centre of the TTX plate. Excess water surrounding the animals was removed with tissue paper Kim-wipe (NIPPON PAPER CRECIA) within 20 s. After 60 min, the animals were killed by chloroform gas, and the animals in each of the eight regions were scored. Auto-tracking system Movements of individual animals were recorded with our custom-made tracking and live imaging systems. Well-fed single animals were placed on a TTX plate for all tracking experiments. An ordinal analog video camera (Olympus) captured freely moving individual animals for 50 min using an adequate sampling rate (30 frames per s). A computer-controlled microscope stage was automatically moved to place an animal at the centre in the visual field using a custom image analysis algorithm within the microscope software MetaMorph (Universal Imaging). The X–Y position of animals on the temperature gradient was measured and recorded once every second using a custom-made algorithm in MetaMorph. In vivo calcium imaging and membrane voltage imaging Well-fed animals expressing yellow cameleon 3.60 driven by the gcy-8, AIY or the ceh-36short promoters, gcy-8p::yc3.60 (pSAS309), AIYp::yc3.60 (pNR86.79) or ceh-36shortp::yc3.60 , respectively, were tested for calcium imaging. Well-fed animals expressing mermaid driven by the gcy-8 promoters, gcy-8p::mermaid (pAK202), were tested for membrane voltage imaging. Animals were glued onto a 2% agar pad on glass, immersed in M9 buffer, and covered by cover glass. The agar pad and M9 buffer were kept at the initial imaging temperature. Sample preparation was completed within 1 min. The sample was then placed onto a peltier-based thermocontroller (Tokai Hit) on the stage of Olympus BX61WI at the initial imaging temperature for 2 min, and fluorescence was introduced into a Dual-View (Molecular devices) optics systems. Fluorescence images of donor and acceptor fluorescent protein in yellow cameleon or mermaid were simultaneously captured by EM-CCD camera C9100-13 ImagEM (Hamamatsu Photonics). Images were taken with a 500-ms exposure time with 1×1 binning. The temperature on the agar pad was monitored by a thermometer system, DCM-20 (Tokai Hit and Hamamatsu Photonics). For each imaging experiment, fluorescence intensities were measured using the MetaMorph (Molecular Device) imaging analysis system. Relative changes in the intracellular calcium concentration or the membrane voltage were measured as changes in the Acceptor/Donor fluorescence ratio of each indicator protein (Ratio change). All band pass filters for experiments using yellow cameleon ( Supplementary Fig. S5a,c ) or mermaid ( Supplementary Fig. S5a,d ) are described in Supplementary Figure S5a,c,d . Activation of halorhodopsin or channelrhodopsin Millisecond scale pulsed-light system using the galvano mirror that allows Hz-controllable deliveries of the excitation light for halorhodopsin and channelrhodopsin was used (GALVANOSHUTTER, Olympus) ( Supplementary Note 1 , Supplementary Figs S1a,c and S5a,b ). In the system, pulse generator SG4115 (IWATSU) was utilized to control pattern of illumination. All band pass filters and mirrors are described in Supplementary Figure S5 . Germline transformation Germline transformations were performed with co-injection mixes consisting of experimental DNA at various concentrations (30–130 ng per microliter) and pNAS88 ges-1p::nls-tag rfp (50 ng per microliter) as a transgenic marker. Molecular biology We optimized the pattern of codon of bacteria halorhodopsin gene ( nphr ) and channelrhodopsin gene ( chr2 ) to that of C. elegans , because of unstable expression of the original bacterial genes in head neurons in C. elegans . The plasmids, pAK222 gcy-8p::CeNpHR-tagRFP and pAK231 gcy-8p::CeNpHR-HcRed , contain codon-optimized halorhodopsin gene ( CeNpHR) fused with a gene encoding red fluorescent protein tagRFP and HcRed, respectively. pAK231 was used specifically in the experiment for membrane voltage imaging. A plasmid, pSHI019 gcy-8p::CeChR2-GFP , contains codon-optimized channelrhodopsin gene ( Ce ChR2) fused with a gene encoding green fluorescent protein (GFP). gcy-8p drives gene expression in AFD thermosensory neuron specifically, as previously reported [4] . Statistical analysis All error bars in the figures indicate standard error of mean (s.e.m.). The statistical analyses for behavioural experiments were performed by one-way analysis of variance (ANOVAs) for multiple comparisons, which were followed by Dunnet post hoc tests. A single asterisk (*), double asterisk (**), and not significant (NS) in the figures indicate P <0.05, P <0.01, and P >0.05, respectively. P means probability. How to cite this article: Kuhara, A. et al . Neural coding in a single sensory neuron controlling opposite seeking behaviors in Caenorhabditis elegans . Nat. Commun. 2:355 doi: 10.1038/ncomms1352 (2011).